Direct measurement of the upper critical field in cuprate superconductors In the quest to increase the critical temperature T c of cuprate superconductors, it is essential to identify the factors that limit the strength of superconductivity. The upper critical field H c2 is a fundamental measure of that strength, yet there is no agreement on its magnitude and doping dependence in cuprate superconductors. Here we show that the thermal conductivity can be used to directly detect H c2 in the cuprates YBa 2 Cu 3 O y , YBa 2 Cu 4 O 8 and Tl 2 Ba 2 CuO 6+ δ , allowing us to map out H c2 across the doping phase diagram. It exhibits two peaks, each located at a critical point where the Fermi surface of YBa 2 Cu 3 O y is known to undergo a transformation. Below the higher critical point, the condensation energy, obtained directly from H c2 , suffers a sudden 20-fold collapse. This reveals that phase competition—associated with Fermi-surface reconstruction and charge-density-wave order—is a key limiting factor in the superconductivity of cuprates. In a type-II superconductor at T =0, the onset of the superconducting state as a function of decreasing magnetic field H occurs at the upper critical field H c2 , dictated by the pairing gap Δ through the coherence length ξ 0 ~ v F /Δ, via H c2 =Φ 0 /2πξ 0 2 , where v F is the Fermi velocity and Φ 0 is the magnetic flux quantum. H c2 is the field below which vortices appear in the sample. Typically, the vortices immediately form a lattice (or solid) and thus cause the electrical resistance to go to zero. So the vortex-solid melting field, H vs , is equal to H c2 . In cuprate superconductors, the strong 2D character and low superfluid density cause a vortex liquid phase to intervene between the vortex-solid phase below H vs ( T ) and the normal state above H c2 ( T ) (ref. 1 ). It has been argued that in underdoped cuprates there is a wide vortex-liquid phase even at T =0 (refs 2 , 3 , 4 , 5 ), so that H c2 (0)>> H vs (0), implying that Δ is very large. Whether the gap Δ is large or small in the underdoped regime is a pivotal issue for understanding what controls the strength of superconductivity in cuprates. So far, however, no measurement on a cuprate superconductor has revealed a clear transition at H c2 , so there are only indirect estimates [2] , [6] , [7] and these vary widely (see Supplementary Discussion and Supplementary Fig. 1 ). For example, superconducting signals in the Nernst effect [2] and the magnetization [4] have been tracked to high fields, but it is difficult to know whether these are due to vortex-like excitations below H c2 or to fluctuations above H c2 (ref. 7 ). Here we demonstrate that measurements of the thermal conductivity can directly detect H c2 , and we show that in the cuprate superconductors YBa 2 Cu 3 O y (YBCO) and YBa 2 Cu 4 O 8 (Y124) there is no vortex liquid at T =0. This fact allows us to then use measurements of the resistive critical field H vs ( T ) to obtain H c2 in the T =0 limit. By including measurements on the overdoped cuprate Tl 2 Ba 2 CuO 6+δ (Tl-2201), we establish the full doping dependence of H c2 . The magnitude of H c2 is found to undergo a sudden drop as the doping is reduced below p =0.18, revealing the presence of a T =0 critical point below which a competing phase markedly weakens superconductivity. This phase is associated with the onset of Fermi-surface reconstruction and charge-density-wave order, generic properties of hole-doped cuprates. Thermal conductivity To detect H c2 , we use the fact that electrons are scattered by vortices, and monitor their mobility as they enter the superconducting state by measuring the thermal conductivity κ of a sample as a function of magnetic field H . In Fig. 1 , we report our data on YBCO and Y124, as κ vs H up to 45 T, at two temperatures well below T c (see Methods and Supplementary Note 1 ). All curves exhibit the same rapid drop below a certain critical field. This is precisely the behaviour expected of a clean type-II superconductor ( l 0 >>ξ 0 ), whereby the long electronic mean free path l 0 in the normal state is suddenly curtailed when vortices appear in the sample and scatter the electrons (see Supplementary Note 2 ). This effect is observed in any clean type-II superconductor, as illustrated in Fig. 1e and Supplementary Fig. 2 . Theoretical calculations [8] reproduce well the rapid drop of κ at H c2 ( Fig. 1e ). 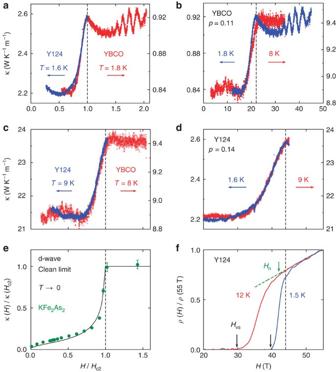Figure 1: Thermal conductivity of YBCO and Y124. (a–d) Magnetic field dependence of the thermal conductivity κ in YBCO (p=0.11) and Y124 (p=0.14), for temperatures as indicated. The end of the rapid rise marks the end of the vortex state, defining the upper critical fieldHc2(vertical dashed line). InFig. 1a,c, the data are plotted as κ vsH/Hc2, withHc2=22 T for YBCO andHc2=44 T for Y124. The remarkable similarity of the normalized curves demonstrates the good reproducibility across dopings. The large quantum oscillations seen in the YBCO data aboveHc2confirm the long electronic mean path in this sample. InFig. 1b,d, the overlap of the two isotherms plotted as κ vsHshows thatHc2(T) is independent of temperature in both YBCO and Y124, up to at least 8 K. (e) Thermal conductivity of the type-II superconductor KFe2As2in theT=0 limit, for a sample in the clean limit (green circles). Error bars represent the uncertainty in extrapolating κ/TtoT=0. The data9are compared with a theoretical calculation for ad-wave superconductor in the clean limit8. (f) Electrical resistivity of Y124 atT=1.5 K (blue) andT=12 K (red) (ref.11). The green arrow defines the fieldHnbelow which the resistivity deviates from its normal-state behaviour (green dashed line). WhileHc2(T) is essentially constant up to 10 K (Fig. 1d),Hvs(T)—the onset of the vortex-solid phase of zero resistance (black arrows)—moves down rapidly with temperature (see alsoFig. 3b). Figure 1: Thermal conductivity of YBCO and Y124. ( a – d ) Magnetic field dependence of the thermal conductivity κ in YBCO ( p =0.11) and Y124 ( p =0.14), for temperatures as indicated. The end of the rapid rise marks the end of the vortex state, defining the upper critical field H c2 (vertical dashed line). In Fig. 1a,c , the data are plotted as κ vs H / H c2 , with H c2 =22 T for YBCO and H c2 =44 T for Y124. The remarkable similarity of the normalized curves demonstrates the good reproducibility across dopings. The large quantum oscillations seen in the YBCO data above H c2 confirm the long electronic mean path in this sample. In Fig. 1b,d , the overlap of the two isotherms plotted as κ vs H shows that H c2 ( T ) is independent of temperature in both YBCO and Y124, up to at least 8 K. ( e ) Thermal conductivity of the type-II superconductor KFe 2 As 2 in the T =0 limit, for a sample in the clean limit (green circles). Error bars represent the uncertainty in extrapolating κ/ T to T =0. The data [9] are compared with a theoretical calculation for a d -wave superconductor in the clean limit [8] . ( f ) Electrical resistivity of Y124 at T =1.5 K (blue) and T =12 K (red) (ref. 11 ). The green arrow defines the field H n below which the resistivity deviates from its normal-state behaviour (green dashed line). While H c2 ( T ) is essentially constant up to 10 K ( Fig. 1d ), H vs ( T )—the onset of the vortex-solid phase of zero resistance (black arrows)—moves down rapidly with temperature (see also Fig. 3b ). Full size image To confirm our interpretation that the drop in κ is due to vortex scattering, we measured a single crystal of Tl-2201 for which l 0 ~ξ 0 , corresponding to a type-II superconductor in the dirty limit. As seen in Fig. 2a , the suppression of κ upon entering the vortex state is much more gradual than in the ultraclean YBCO. The contrast between Tl-2201 and YBCO mimics the behaviour of the type-II superconductor KFe 2 As 2 as the sample goes from clean ( l 0 ~10 ξ 0 ) (ref. 9 ) to dirty ( l 0 ~ξ 0 ) (ref. 10 ) (see Fig. 2b ). We conclude that the onset of the sharp drop in κ with decreasing H in YBCO is a direct measurement of the critical field H c2 , where vortex scattering begins. 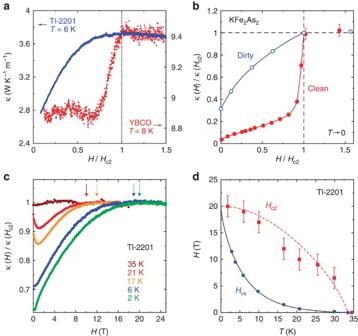Figure 2: Thermal conductivity andH-Tdiagram of Tl-2201. (a) Magnetic field dependence of the thermal conductivity κ in Tl-2201, measured atT=6 K on an overdoped sample withTc=33 K (blue). The data are plotted as κ vsH/Hc2, withHc2=19 T, and compared with data on YBCO atT=8 K (red; fromFig. 1b), withHc2=23 T. (b) Corresponding data for KFe2As2, taken on clean9(red) and dirty10(blue) samples. (c) Isotherms of κ(H) in Tl-2201, at temperatures as indicated, where κ is normalized to unity atHc2(arrows).Hc2is defined as the field below which κ starts to fall with decreasing field. (d) Temperature dependence ofHc2(red squares) andHvs(blue circles) in Tl-2201. Error bars on theHc2data represent the uncertainty in locating the onset of the drop in κ vsHrelative to the constant normal-state behaviour. All lines are a guide to the eye. Figure 2: Thermal conductivity and H - T diagram of Tl-2201. ( a ) Magnetic field dependence of the thermal conductivity κ in Tl-2201, measured at T =6 K on an overdoped sample with T c =33 K (blue). The data are plotted as κ vs H / H c2 , with H c2 =19 T, and compared with data on YBCO at T =8 K (red; from Fig. 1b ), with H c2 =23 T. ( b ) Corresponding data for KFe 2 As 2 , taken on clean [9] (red) and dirty [10] (blue) samples. ( c ) Isotherms of κ( H ) in Tl-2201, at temperatures as indicated, where κ is normalized to unity at H c2 (arrows). H c2 is defined as the field below which κ starts to fall with decreasing field. ( d ) Temperature dependence of H c2 (red squares) and H vs (blue circles) in Tl-2201. Error bars on the H c2 data represent the uncertainty in locating the onset of the drop in κ vs H relative to the constant normal-state behaviour. All lines are a guide to the eye. Full size image Upper critical field H c2 The direct observation of H c2 in a cuprate material is our first main finding. We obtain H c2 =22±2 T at T =1.8 K in YBCO (at p =0.11) and H c2 =44±2 T at T =1.6 K in Y124 (at p =0.14) ( Fig. 1a ), giving ξ 0 =3.9 nm and 2.7 nm, respectively. In Y124, the transport mean free path l 0 was estimated to be roughly 50 nm (ref. 11 ), so that the clean-limit condition l 0 >>ξ 0 is indeed satisfied. Note that the specific heat is not sensitive to vortex scattering and so will have a much less pronounced anomaly at H c2 . This is consistent with the high-field specific heat of YBCO at p =0.1 (ref. 5 ). We can verify that our measurement of H c2 in YBCO is consistent with existing thermodynamic and spectroscopic data by computing the condensation energy δE = H c 2 /2μ 0 , where H c 2 = H c1 H c2 /(ln κ GL +0.5), with H c1 the lower critical field and κ GL the Ginzburg-Landau parameter (ratio of penetration depth to coherence length). Magnetization data [12] on YBCO give H c1 =24±2 mT at T c =56 K. Using κ GL =50 (ref. 12 ), our value of H c2 =22 T (at T c =61 K) yields δE / T c 2 =13±3 J K −2 m −3 . For a d -wave superconductor, δE = N F Δ 0 2 /4, where Δ 0 =α k B T c is the gap maximum and N F is the density of states at the Fermi energy, related to the electronic specific heat coefficient γ N =(2π 2 /3) N F k B 2 , so that δE / T c 2 =(3α 2 /8π 2 ) γ N . Specific heat data [5] on YBCO at T c =59 K give γ N =4.5±0.5 mJ K −2 mol −1 (43±5 J /K −2 m −3 ) above H c2 . We therefore obtain α=2.8±0.5, in good agreement with estimates from spectroscopic measurements on a variety of hole-doped cuprates, which yield 2Δ 0 / k B T c ~5 between p =0.08 and p =0.24 (ref. 13 ). This shows that the value of H c2 measured by thermal conductivity provides quantitatively coherent estimates of the condensation energy and gap magnitude in YBCO. H — T phase diagram The position of the rapid drop in κ vs H does not shift appreciably with temperature up to T ~10 K or so ( Fig. 1b,d ), showing that H c2 ( T ) is essentially flat at low temperature. This is in sharp contrast with the resistive transition at H vs ( T ), which moves down rapidly with increasing temperature ( Fig. 1f ). In Fig. 3 , we plot H c2 ( T ) and H vs ( T ) on an H - T diagram, for both YBCO and Y124 (see Methods and Supplementary Methods ). In both cases, we see that H c2 = H vs in the T =0 limit. This is our second main finding: there is no vortex liquid regime at T =0 (see Supplementary Note 3 ). With increasing temperature the vortex-liquid phase grows rapidly, causing H vs ( T ) to fall below H c2 ( T ). The same behaviour is seen in Tl-2201 ( Fig. 2d ): at low temperature, H c2 ( T ) determined from κ is flat, whereas H vs ( T ) from resistivity falls abruptly, and H c2 = H vs at T →0 (see also Supplementary Figs 3 and 4 , and Supplementary Note 4 ). 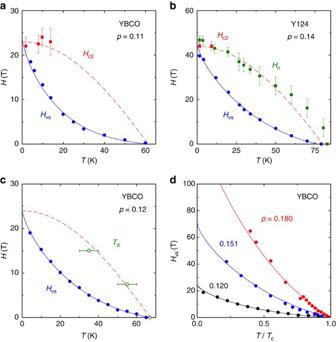Figure 3: Field-temperature phase diagram of YBCO and Y124. (a,b) Temperature dependence ofHc2(red squares, from data as inFig. 1) for YBCO and Y124, respectively. The red dashed line is a guide to the eye, showing howHc2(T) might extrapolate to zero atTc. Error bars on theHc2data represent the uncertainty in locating the onset of the downward deviation in κ vsHrelative to the normal-state behaviour. The solid lines are a fit of theHvs(T) data (solid circles) to the theory of vortex-lattice melting1, as in ref.14. Note thatHc2(T) andHvs(T) converge atT=0, in both materials, so that measurements ofHvsvsTcan be used to determineHc2(0). InFig. 3b, we plot the fieldHndefined inFig. 1f(open green squares, from data in ref.11), which corresponds roughly to the upper boundary of the vortex-liquid phase (seeSupplementary Note 3). Error bars on theHndata represent the uncertainty in locating the onset of the downward deviation in ρ vsHrelative to the normal-state behaviour. We see thatHn(T) is consistent withHc2(T). (c) TemperatureTXbelow which charge order is suppressed by the onset of superconductivity in YBCO atp=0.12, as detected by X-ray diffraction24(open green circles, fromSupplementary Fig. 7). Error bars on theTXdata represent the uncertainty in locating the onset of the downward deviation in the x-ray intensity vsTat a given field relative to the data at 17 T (seeSupplementary Fig. 7a). We see thatTX(H) follows a curve (red dashed line) that is consistent withHn(T) (atp=0.14;Fig. 3b) and with theHc2(T) detected by thermal conductivity at lower temperature (atp=0.11 and 0.14). (d)Hvs(T) vsT/Tc, showing a marked increase inHvs(0) aspgoes from 0.12 to 0.18. From these and other data (inSupplementary Fig. 6), we obtain theHvs(T→0) values that produce theHc2vspcurve plotted inFig. 4a. Figure 3: Field-temperature phase diagram of YBCO and Y124. ( a , b ) Temperature dependence of H c2 (red squares, from data as in Fig. 1 ) for YBCO and Y124, respectively. The red dashed line is a guide to the eye, showing how H c2 ( T ) might extrapolate to zero at T c . Error bars on the H c2 data represent the uncertainty in locating the onset of the downward deviation in κ vs H relative to the normal-state behaviour. The solid lines are a fit of the H vs ( T ) data (solid circles) to the theory of vortex-lattice melting [1] , as in ref. 14 . Note that H c2 ( T ) and H vs ( T ) converge at T =0, in both materials, so that measurements of H vs vs T can be used to determine H c2 (0). In Fig. 3b , we plot the field H n defined in Fig. 1f (open green squares, from data in ref. 11 ), which corresponds roughly to the upper boundary of the vortex-liquid phase (see Supplementary Note 3 ). Error bars on the H n data represent the uncertainty in locating the onset of the downward deviation in ρ vs H relative to the normal-state behaviour. We see that H n ( T ) is consistent with H c2 ( T ). ( c ) Temperature T X below which charge order is suppressed by the onset of superconductivity in YBCO at p =0.12, as detected by X-ray diffraction [24] (open green circles, from Supplementary Fig. 7 ). Error bars on the T X data represent the uncertainty in locating the onset of the downward deviation in the x-ray intensity vs T at a given field relative to the data at 17 T (see Supplementary Fig. 7a ). We see that T X ( H ) follows a curve (red dashed line) that is consistent with H n ( T ) (at p =0.14; Fig. 3b ) and with the H c2 ( T ) detected by thermal conductivity at lower temperature (at p =0.11 and 0.14). ( d ) H vs ( T ) vs T / T c , showing a marked increase in H vs (0) as p goes from 0.12 to 0.18. From these and other data (in Supplementary Fig. 6 ), we obtain the H vs ( T →0) values that produce the H c2 vs p curve plotted in Fig. 4a . Full size image H — p phase diagram Having established that H c2 = H vs at T →0 in YBCO, Y124 and Tl-2201, we can determine how H c2 varies with doping from measurements of H vs ( T ) (see Methods and Supplementary Methods ), as in Supplementary Figs 5 and 6 . For p <0.15, fields lower than 60 T are sufficient to suppress T c to zero, and thus directly assess H vs ( T →0), yielding H c2 =24±2 T at p =0.12 ( Fig. 3c ), for example. For p >0.15, however, T c cannot be suppressed to zero with our maximal available field of 68 T ( Fig. 3d and Supplementary Fig. 5 ), so an extrapolation procedure must be used to extract H vs ( T →0). Following ref. 14 , we obtain H vs ( T →0) from a fit to the theory of vortex-lattice melting [1] , as illustrated in Fig. 3 (and Supplementary Fig. 6 ). In Fig. 4a , we plot the resulting H c2 values as a function of doping, listed in Table 1 , over a wide doping range from p =0.05 to p =0.26. This brings us to our third main finding: the H — p phase diagram of superconductivity consists of two peaks, located at p 1 ~0.08 and p 2 ~0.18. (A partial plot of H vs ( T →0) vs p was reported earlier on the basis of c -axis resistivity measurements [14] , in excellent agreement with our own results.) The two-peak structure is also apparent in the usual T — p plane: the single T c dome at H =0 transforms into two domes when a magnetic field is applied ( Fig. 4b ). 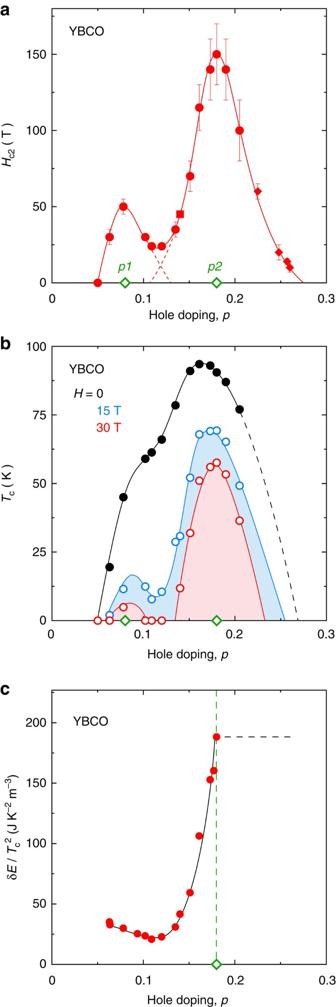Figure 4: Doping dependence ofHc2,Tcand the condensation energy. (a) Upper critical fieldHc2of the cuprate superconductor YBCO as a function of hole concentration (doping)p.Hc2is defined asHvs(T→0) (Table 1), the onset of the vortex-solid phase atT→0, whereHvs(T) is obtained from high-field resistivity data (Fig. 3, andSupplementary Figs 5 and 6). The point atp=0.14 (square) is from data on Y124 (Fig. 3b). The points atp>0.22 (diamonds) are from data on Tl-2201 (Table 1,Fig. 2andSupplementary Fig. 6). Error bars on theHc2data represent the uncertainty in extrapolating theHvs(T) data toT=0. (b) Critical temperatureTcof YBCO as a function of dopingp, for three values of the magnetic fieldH, as indicated (Table 1).Tcis defined as the point of zero resistance. All lines are a guide to the eye. Two peaks are observed inHc2(p) and inTc(p;H>0), located atp1~0.08 andp2~0.18 (open diamonds). The first peak coincides with the onset of incommensurate spin modulations atp≈0.08, detected by neutron scattering30and muon spin spectroscopy31. The second peak coincides with the approximate onset of Fermi-surface reconstruction18,21, attributed to charge modulations detected by high-field NMR (ref.22) and X-ray scattering23,24,25. (c) Condensation energy δE(red circles), given by the product ofHc2andHc1(seeSupplementary Note 5andSupplementary Fig. 8), plotted as δE/Tc2vsp. Note the eightfold drop belowp2(vertical dashed line), attributed predominantly to a corresponding drop in the density of states. All lines are a guide to the eye. Figure 4: Doping dependence of H c2 , T c and the condensation energy. ( a ) Upper critical field H c2 of the cuprate superconductor YBCO as a function of hole concentration (doping) p . H c2 is defined as H vs ( T →0) ( Table 1 ), the onset of the vortex-solid phase at T →0, where H vs ( T ) is obtained from high-field resistivity data ( Fig. 3 , and Supplementary Figs 5 and 6 ). The point at p =0.14 (square) is from data on Y124 ( Fig. 3b ). The points at p >0.22 (diamonds) are from data on Tl-2201 ( Table 1 , Fig. 2 and Supplementary Fig. 6 ). Error bars on the H c2 data represent the uncertainty in extrapolating the H vs ( T ) data to T =0. ( b ) Critical temperature T c of YBCO as a function of doping p , for three values of the magnetic field H , as indicated ( Table 1 ). T c is defined as the point of zero resistance. All lines are a guide to the eye. Two peaks are observed in H c2 ( p ) and in T c ( p ; H >0), located at p 1 ~0.08 and p 2 ~0.18 (open diamonds). The first peak coincides with the onset of incommensurate spin modulations at p ≈0.08, detected by neutron scattering [30] and muon spin spectroscopy [31] . The second peak coincides with the approximate onset of Fermi-surface reconstruction [18] , [21] , attributed to charge modulations detected by high-field NMR (ref. 22 ) and X-ray scattering [23] , [24] , [25] . ( c ) Condensation energy δ E (red circles), given by the product of H c2 and H c1 (see Supplementary Note 5 and Supplementary Fig. 8 ), plotted as δ E / T c 2 vs p . Note the eightfold drop below p 2 (vertical dashed line), attributed predominantly to a corresponding drop in the density of states. All lines are a guide to the eye. Full size image Table 1 Samples used in resistance measurements. Full size table A natural explanation for two peaks in the H c2 vs p curve is that each peak is associated with a distinct critical point where some phase transition occurs. An example of this is the heavy-fermion metal CeCu 2 Si 2 , where two T c domes in the temperature-pressure phase diagram were revealed by adding impurities to weaken superconductivity [15] : one dome straddles an underlying antiferromagnetic transition and the other dome a valence transition [16] . In YBCO, there is indeed strong evidence of two transitions—one at p 1 and another at a critical doping consistent with p 2 (ref. 17 ). In particular, the Fermi surface of YBCO is known to undergo one transformation at p =0.08 and another near p ~0.18 (ref. 18 ). Hints of two critical points have also been found in Bi 2 Sr 2 CaCu 2 O 8+δ , as changes in the superconducting gap detected by ARPES at p 1 ~0.08 and p 2 ~0.19 (ref. 19 ). The transformation at p 2 is a reconstruction of the large hole-like cylinder at high doping that produces a small electron pocket [18] , [20] , [21] . We associate the fall of T c and the collapse of H c2 below p 2 to that Fermi-surface reconstruction. Recent studies indicate that charge-density wave order plays a role in the reconstruction [22] , [23] , [24] , [25] . Indeed, the charge modulation seen with X-rays [23] , [24] , [25] and the Fermi-surface reconstruction seen in the Hall coefficient [18] , [26] emerge in parallel with decreasing temperature (see Fig. 5 ). Moreover, the charge modulation amplitude drops suddenly below T c , showing that superconductivity and charge order compete [23] , [24] , [25] ( Supplementary Fig. 7a ). As a function of field [24] , the onset of this competition defines a line in the H — T plane ( Supplementary Fig. 7b ) that is consistent with our H c2 ( T ) line ( Fig. 3 ). The flip side of this phase competition is that superconductivity must in turn be suppressed by charge order, consistent with our interpretation of the T c fall and H c2 collapse below p 2 . 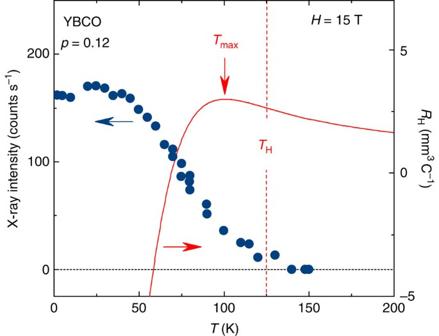Figure 5: Fermi-surface reconstruction and charge order. Hall coefficientRH(T) of YBCO as a function of temperature at a dopingp=0.12 (Tc=66 K), for a fieldH=15 T (red line, from ref.26).Tmaxis the temperature at which the Hall coefficientRH(T) peaks, before it falls to reach negative values—a signature of Fermi-surface reconstruction18,21.THis the inflexion point where the downturn inRH(T) begins. The evolution ofRH(T) is compared with the growth of charge-density-wave modulations in YBCO detected by X-ray diffraction, at the same doping and field24. As seen, the onset of the modulations, atTCO~130 K, coincides withTH. This suggests a causal connection between charge order and Fermi-surface reconstruction. Figure 5: Fermi-surface reconstruction and charge order. Hall coefficient R H ( T ) of YBCO as a function of temperature at a doping p =0.12 ( T c =66 K), for a field H =15 T (red line, from ref. 26 ). T max is the temperature at which the Hall coefficient R H ( T ) peaks, before it falls to reach negative values—a signature of Fermi-surface reconstruction [18] , [21] . T H is the inflexion point where the downturn in R H ( T ) begins. The evolution of R H ( T ) is compared with the growth of charge-density-wave modulations in YBCO detected by X-ray diffraction, at the same doping and field [24] . As seen, the onset of the modulations, at T CO ~130 K, coincides with T H . This suggests a causal connection between charge order and Fermi-surface reconstruction. Full size image We can quantify the impact of phase competition by computing the condensation energy δE at p = p 2 , using H c1 =110±5 mT at T c =93 K (ref. 27 ) and H c2 =140±20 T ( Table 1 ), and comparing with δE at p =0.11 (see above): δE decreases by a factor 20 and δE / T c 2 by a factor 8 (see Supplementary Note 5 ). In Fig. 4c , we plot the doping dependence of δE / T c 2 (in qualitative agreement with earlier estimates based on specific heat data [28] —see Supplementary Fig. 8 ). We attribute the tremendous weakening of superconductivity below p 2 to a major drop in the density of states as the large hole-like Fermi surface reconstructs into small pockets. This process is likely to involve both the pseudogap formation and the charge ordering. Upon crossing below p =0.08, the Fermi surface of YBCO undergoes a second transformation, where the small electron pocket disappears, signalled by pronounced changes in transport properties [18] , [21] and in the effective mass m * (ref. 29 ). This is strong evidence that the peak in H c2 at p 1 ~0.08 ( Fig. 4a ) coincides with an underlying critical point. This critical point is presumably associated with the onset of incommensurate spin modulations detected below p ~0.08 by neutron scattering [30] and muon spectroscopy [31] . Note that the increase in m * (ref. 29 ) may in part explain the increase in H c2 going from p =0.11 (local minimum) to p =0.08, since H c2 ~1/ξ 0 2 ~1/ v F 2 ~ m *2 . Our findings shed light on the H - T - p phase diagram of cuprate superconductors, in three different ways. In the H - p plane, they establish the boundary of the superconducting phase and reveal a two-peak structure, the likely fingerprint of two underlying critical points. In the H - T plane, they delineate the separate boundaries of vortex solid and vortex liquid phases, showing that the latter phase vanishes as T →0. In the T - p plane, they elucidate the origin of the dome-like T c curve as being primarily due to phase competition, rather than fluctuations in the phase of the superconducting order parameter [32] , and they quantify the impact of that competition on the condensation energy. Our finding of a collapse in condensation energy due to phase competition is likely to be a generic property of hole-doped cuprates, since Fermi-surface reconstruction—the inferred cause—has been observed in materials such as La 1.8 -x Eu 0.2 Sr x CuO 4 (ref. 20 ) and HgBa 2 CuO 4 +δ (refs 33 , 34 ), two cuprates whose structure is significantly different from that of YBCO and Y124. This shows that phase competition is one of the key factors that limit the strength of superconductivity in high- T c cuprates. Samples Single crystals of YBa 2 Cu 3 O y (YBCO) were obtained by flux growth at UBC (ref. 35 ). The superconducting transition temperature T c was determined as the temperature below which the zero-field resistance R =0. The hole doping p is obtained from T c (ref. 36 ). To access dopings above p =0.18, Ca substitution was used, at the level of 1.4% (giving p =0.19) and 5% (giving p =0.205). At oxygen content y =6.54, a high degree of ortho-II oxygen order has been achieved, yielding large quantum oscillations [37] , [38] , proof of a long electronic mean free path. We used such crystals for our thermal conductivity measurements. Single crystals of YBa 2 Cu 4 O 8 (Y124) were grown by a flux method in Y 2 O 3 crucibles and an Ar/O 2 mixture at 2,000 bar, with a partial oxygen pressure of 400 bar (ref. 39 ). Y124 is a stoichiometric underdoped cuprate material, with T c =80 K. The doping is estimated from the value of T c , using the same relation as for YBCO (ref. 36 ). Because of its high intrinsic level of oxygen order, quantum oscillations have also been observed in the highest quality crystals of Y124 (ref. 40 ). We used such crystals for our thermal conductivity measurements. Single crystals of Tl 2 Ba 2 CuO 6 (Tl-2201) were obtained by flux growth at UBC. Compared with YBCO and Y124, crystals of Tl-2201 are in the dirty limit (see Supplementary Note 4 ). We used such crystals to compare thermal conductivity data in the clean and dirty limits. The thermal conductivity (and resistivity) was measured on two strongly overdoped samples of Tl-2201 with T c =33 K and 20 K, corresponding to a hole doping p =0.248 and 0.257, respectively. The doping value for Tl-2201 samples was obtained from their T c , via the standard formula T c / T c max =1–82.6 ( p –0.16) 2 , with T c max =90 K. Resistivity measurements The in-plane electrical resistivity of YBCO was measured in magnetic fields up to 45 T at the NHMFL in Tallahassee and up to 68 T at the LNCMI in Toulouse. A subset of those data is displayed in Supplementary Fig. 5 . From such data, H vs ( T ) is determined and extrapolated to T =0 to get H vs (0), as illustrated in Fig. 3 and Supplementary Fig. 6 . The H c2 = H vs (0) values thus obtained are listed in Table 1 and plotted in Fig. 4a . Corresponding data on Y124 were taken from ref. 11 (see Supplementary Fig. 5 ). The resistance of a Tl-2201 sample with T c =59 K ( p =0.225) was also measured, at the LNCMI in Toulouse up to 68 T (see Supplementary Figs 5 and 6 ). In all measurements, the magnetic field was applied along the c axis, normal to the CuO 2 planes. (See also Supplementary Methods .) Thermal conductivity measurements The thermal conductivity κ of four ortho-II oxygen-ordered samples of YBCO, with p =0.11, was measured at the LNCMI in Grenoble up to 34 T and/or at the NHMFL in Tallahassee up to 45 T, in the temperature range from 1.8 K to 14 K. Data from the four samples were in excellent agreement (see Table 2 ). The thermal conductivity κ of two single crystals of stoichiometric Y124 ( p =0.14) was measured at the NHMFL in Tallahassee up to 45 T, in the temperature range from 1.6 K to 9 K. Data from the two samples were in excellent agreement (see Table 2 ). Table 2 Samples used in thermal conductivity measurements. Full size table A constant heat current Q was sent in the basal plane of the single crystal, generating a thermal gradient d T across the sample. The thermal conductivity is defined as κ=( Q /d T ) ( L / w t ), where L , w and t are the length (across which d T is measured), width and thickness (along the c axis) of the sample, respectively. The thermal gradient d T = T hot − T cold was measured with two Cernox thermometers, sensing the temperature at the hot ( T hot ) and cold ( T cold ) ends of the sample, respectively. The Cernox thermometers were calibrated by performing field sweeps at different closely spaced temperatures between 2 K and 15 K. Representative data are shown in Fig. 1 . (See also Supplementary Note 1 .) How to cite this article: Grissonnanche, G. et al . Direct measurement of the upper critical field in cuprate superconductors. Nat. Commun. 5:3280 doi: 10.1038/ncomms4280 (2014).